Bacterial twitching motility is coordinated by a two-dimensional tug-of-war with directional memory Type IV pili are ubiquitous bacterial motors that power surface motility. In peritrichously piliated species, it is unclear how multiple pili are coordinated to generate movement with directional persistence. Here we use a combined theoretical and experimental approach to test the hypothesis that multiple pili of Neisseria gonorrhoeae are coordinated through a tug-of-war. Based on force-dependent unbinding rates and pilus retraction speeds measured at the level of single pili, we build a tug-of-war model. Whereas the one-dimensional model robustly predicts persistent movement, the two-dimensional model requires a mechanism of directional memory provided by re-elongation of fully retracted pili and pilus bundling. Experimentally, we confirm memory in the form of bursts of pilus retractions. Bursts are seen even with bundling suppressed, indicating re-elongation from stable core complexes as the key mechanism of directional memory. Directional memory increases the surface range explored by motile bacteria and likely facilitates surface colonization. Mechanical forces generated in cells and by cells influence many biological processes such as intracellular transport and structure formation, cell division, cell motility and tissue development [1] , [2] , [3] , [4] , [5] . Force generation depends on molecular motors, which often act cooperatively to generate forces exceeding the single-motor forces [6] , [7] . How cooperative motors are coordinated is an area of active research. Studies on transport by cytoskeletal motors have shown that a key aspect of such coordination is mechanical in nature: a motor’s dynamical properties are influenced by the forces generated by other motors. In bidirectional cytoskeletal transport, these forces result in a tug-of-war between motors pulling a common cargo in opposing directions. On theoretical grounds a tug-of-war mechanism has been proposed for efficient bidirectional transport [8] and several recent experimental studies on microtubule-based transport support such a mechanism [9] , [10] , [11] (although some studies also provide evidence of additional non-mechanical coordination mechanisms in some systems [12] , [13] ). Likewise, there is evidence supporting a tug-of-war mechanism for oscillations of the mitotic spindle [14] . In all the examples studied so far, a tug-of-war takes place in an essentially one-dimensional situation with motors pulling into opposing directions. In this study, we use a combined theoretical and experimental approach and introduce a two-dimensional tug-of-war model for the twitching motility of Neisseria gonorrhoeae [15] . Twitching is a mechanism for bacterial motility along a surface driven by type IV pili [16] , [17] , [18] , [19] , [20] , micron-sized polymeric cell appendages that play a role not only in motility but also in cell–cell adhesion, cell-surface adhesion and horizontal gene transfer [20] , [21] , [22] . Pili drive motility through cycles of polymerization, adhesion and retraction: When attached to a surface, the retraction of a pilus into the cell body via its depolymerization pulls the bacterium forward along that surface [19] . The dynamics of pilus retraction has been studied extensively [19] , [20] , [23] , [24] . Individual type IV pili generate forces exceeding 100 pN (ref. 25 ). These forces are far larger than the forces generated by other molecular motors, but the velocity of retraction (1–2 μm s −1 ) is in the same range as velocities of cytoskeletal motors. Bundles of pili can generate forces in the nN range [26] . Retraction is dependent on the presence of the PilT protein, an ATPase located at the base of the pilus [27] . The coordination of multiple pili depends on the where pili are located on the cell surface and appears to be different in different bacterial species. In rod-shaped bacteria such as Pseudomonas aeruginosa and Myxococcus xanthus , pili extend from the cell poles, but are usually found only at one pole at a time [19] , [28] . In M. xanthus it has also been shown that the presence of pili at the poles is dynamically regulated through the localized activation of the assembly system (which itself has recently been shown to be stable and remain at both poles [29] ) and clustering of the PilT and PilB proteins, two antagonistic ATPases promoting pilus retraction and elongation, respectively [28] . In both species, the patterns of motion can be complex with several modes of pili-dependent motility in P. aeruginosa [30] , [31] and both pili-dependent and pili-independent mechanisms of surface motility in M. xanthus [32] . By contrast, in spherical bacteria such as N. gonorrhoeae and N. meningitidis pili extend homogeneously in all directions ( Fig. 1a ). No biochemical mechanism coordinating their retraction is known, yet the quantitative analysis of bacterial trajectories provides clear evidence for the cooperation of multiple pili [15] . These observations suggested that the coordination of multiple pilus motors may be mediated mechanically via a tug-of-war of pilus motors pulling in different directions [15] . Furthermore, diplococci (pairs of bacteria) were observed to align and meander in micro-topographic grooves, consistent with a tug-of-war between pili on either side of the bacterium [33] . Moreover, type IV pili fulfil several prerequisites of a tug-of-war mechanism: the persistence time of the motion increases with the number of pili present on the cell surface and the average unbinding force is by an order of magnitude lower than the maximum force that one pilus can generate [15] . The latter feature is a key requirement for a tug-of-war mechanism [8] , and enables pili to pull other pili off the surface. 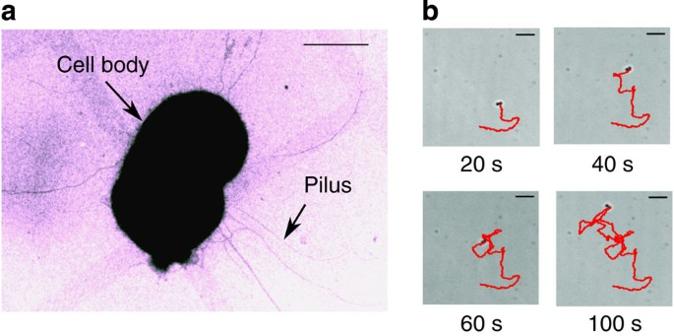Figure 1: Experimental characterization of gonococcal twitching motility. (a) Electron micrograph of aN. gonorrhoeaecell with pili extending in all directions (scale bar, 500 nm). (b) Typical trace of a bacterium moving on a BSA-coated glass surface (scale bar, 5 μm). Figure 1: Experimental characterization of gonococcal twitching motility. ( a ) Electron micrograph of a N. gonorrhoeae cell with pili extending in all directions (scale bar, 500 nm). ( b ) Typical trace of a bacterium moving on a BSA-coated glass surface (scale bar, 5 μm). Full size image In this study, we develop and test a quantitative model for a two-dimensional tug-of-war mechanism, based on the force-dependent properties (unbinding and retraction) measured for single pili. By comparing the theoretical patterns of motility with our previous experiments [15] , we show that bundling of pili or re-elongation of pili that have fully retracted (or both) is required to quantitatively explain the observations. In the absence of both, the directional persistence of the trajectories is underestimated compared with the experiments and the tug-of-war mechanism is less efficient in coordinating the pili. Both features provide a mechanism for directional memory beyond the length of a pilus. As a consequence of directional memory, the retraction events observed in optical tweezers experiments should occur in bursts. We test this prediction experimentally and show that bursts of retractions are indeed observed. Bursts are observed even when bundling of pili is suppressed, indicating re-elongation of pili as the key mechanism of directional memory. Taken together our theoretical and experimental results indicate that bacterial motility driven cooperatively by multiple pili can be explained by a two-dimensional stochastic tug-of-war with directional memory. Quantitative characterization of twitching motility The twitching motility of N. gonorrhoeae cells on glass surfaces has recently been characterized quantitatively [15] . We briefly summarize the main results that are relevant to our present study: The trajectories of bacteria ( Fig. 1b ) exhibit directed motion over times smaller than a persistence time t c and random, effectively diffusive motion for long times. t c is determined by fitting a persistent random walk model to the time-dependence of the mean-square displacement δ 2 ( t ) of the bacteria, δ 2 ( t )= D eff ( t − t c [1−exp(− t / t c )]), where D eff is an effective diffusion constant. Importantly, the distance over which movements are directed was found to exceed the length of a pilus [15] , indicating that motility is based on the cooperation of several pili. In the following, we will refer to the motion as ‘persistent’ if this condition is met, that is, if the persistence length ( L p = t c v r with the retraction velocity v r ) exceeds the pilus length or, equivalently if the persistence time exceeds the time required for the full retraction of a pilus. Moreover, experiments were done with a bacterial strain in which the number of pili per cell could be varied through inducible expression of the pilE gene that encodes the pilus subunit PilE. While the number of pili is modulated by changing the levels of PilE, the length of the pili is essentially unaffected ( Supplementary Table 1 ), as reported previously [15] , [34] . These experiments showed an increase of the persistence time with increasing pilus number [15] . These observations demonstrate that twitching is based on the cooperation between pili. Together with the measurements of the forced rupture of the surface attachment of pili (discussed below) and the absence of evidence supporting a biochemical coordination mechanism of pili, the observations also suggest that the coordination of pili may be mediated mechanically by a tug-of-war between pili that pull into different directions. Force-dependence of unbinding rate and velocity A key feature of mechanical coordination via a tug-of-war mechanism is that the molecular motors involved in the tug-of-war (in our case, the pili) can generate sufficiently large forces to pull other motors off from their track or surface [8] , [35] . This feature is based on a force-dependent unbinding rate ε ( F ) and leads to an instability that amplifies imbalances in the force experienced by motors pulling into opposite directions. Previous experiments indicated that the pili of N. gonorrhoeae satisfy this criterion [15] , but the unbinding rate of the pili from the surface had not been characterized quantitatively. We therefore determined the force-dependence of the unbinding time using an optical trap with force feedback ( Fig. 2a , see also Supplementary Note 1 ). 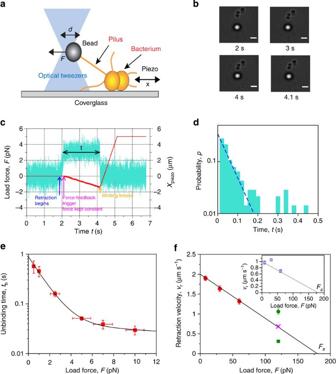Figure 2: Force-dependence of unbinding rate and velocity of individual pili: (a) Setup for characterizing single pilus dynamics (F, force;d, deflection of the bead from the centre of the optical tweezers). (b) Time lapse of two cells (diplococci) and the bead in the laser trap (scale bar, 2 μm). (c) ForceFacting on the bead (turquoise) due to the deflection of the bead from the centre of the laser trap caused by pilus retraction and movements of the piezo stagexpiezo(red). The pilus pulls on the bead until the force feedback is triggered at the preset force of 2.5 pN. The data correspond to the time series shown in (b). (d) Histogram of unbinding times at a force of 5 pN and exponential fit to the data (blue). (e) Characteristic unbinding timetbof individual pili from BSA-coated silica beads as function of the load forceF. The line is a double-exponential fit. Error bars intbindicate s.e. values of the exponential fits as in (d); error bars forFare based on the s.d. of Brownian motion in the laser trap (n>35 for all force values). (f) Force–velocity relation: retraction velocityvrof single pili as a function of the load forceFfor aerobic (red, green) and anaerobic conditions (inset, blue). Data points forF<100 pN are from our previous work48. The green data points at 120 pN (newly measured) correspond to two velocity modes (see alsoSupplementary Fig. 2), the pink cross marks the average velocity for 120 pN, which is used in the model. The lines are linear fits to the data. The error bars indicate s.e. values from averaging overn>20 retractions for each force value. Figure 2: Force-dependence of unbinding rate and velocity of individual pili: ( a ) Setup for characterizing single pilus dynamics ( F , force; d , deflection of the bead from the centre of the optical tweezers). ( b ) Time lapse of two cells (diplococci) and the bead in the laser trap (scale bar, 2 μm). ( c ) Force F acting on the bead (turquoise) due to the deflection of the bead from the centre of the laser trap caused by pilus retraction and movements of the piezo stage x piezo (red). The pilus pulls on the bead until the force feedback is triggered at the preset force of 2.5 pN. The data correspond to the time series shown in ( b ). ( d ) Histogram of unbinding times at a force of 5 pN and exponential fit to the data (blue). ( e ) Characteristic unbinding time t b of individual pili from BSA-coated silica beads as function of the load force F . The line is a double-exponential fit. Error bars in t b indicate s.e. values of the exponential fits as in ( d ); error bars for F are based on the s.d. of Brownian motion in the laser trap ( n >35 for all force values). ( f ) Force–velocity relation: retraction velocity v r of single pili as a function of the load force F for aerobic (red, green) and anaerobic conditions (inset, blue). Data points for F <100 pN are from our previous work [48] . The green data points at 120 pN (newly measured) correspond to two velocity modes (see also Supplementary Fig. 2 ), the pink cross marks the average velocity for 120 pN, which is used in the model. The lines are linear fits to the data. The error bars indicate s.e. values from averaging over n >20 retractions for each force value. Full size image To this end, we approached a BSA-coated silica bead to the bacterium ( Fig. 2a,b ). When pilus retraction started, the bead was pulled out of the centre of the laser trap and thus the force increased steadily. At a preset force, the force feedback was triggered and the distance of the bead from the centre of the trap was maintained constant by moving the sample with a piezo stage ( Fig. 2c ) until the pilus unbound from the bead (for an argument that the observed release corresponds to pilus unbinding rather than breaking, see Supplementary Note 1 and Supplementary Fig. 1 ). For each force value, the distribution of unbinding times was exponential, up to a tail at large forces ( Fig. 2d ). By fitting with an exponential distribution, we obtained the characteristic unbinding time t b ( F ). The unbinding time t b ( F ) was found to exhibit a double-exponential dependence on the force F ( Fig. 2e , see Supplementary Table 2 for the parameters), The force-dependent detachment rate ε ( F ) is then obtained as ε ( F )=1/ t b ( F ). The two characteristic force scales for detachment, F d ,1 =1.28 pN and F d ,2 =33.8 pN, are both smaller than the stall force of pilus retraction ( F s =180 pN, Fig. 2f ), as required for a tug-of-war mechanism. Force–velocity relations are shown in Fig. 2f . The speed of pilus retraction decreases approximately linearly as a function of the external force for both aerobic and anaerobic conditions. At forces below 100 pN, the speed under aerobic conditions is about twofold larger than under anaerobic conditions [36] . At very high force, pilus retraction exhibits stochastic switching between two distinct velocity modes under aerobic conditions (green data points at 120 pN in Fig. 2f , Supplementary Note 2 and Supplementary Fig. 2 ). Speed switching was, however, not included in the model below, where such large forces occur very infrequently (see below). Instead, at large force, we used the average velocity between both modes (the pink cross in Fig. 2f ), extrapolating the linear force–velocity relation to larger forces. The force-dependencies of the unbinding rate and the retraction velocity provide the quantitative description of the dynamics of a single pilus on which the tug-of-war mechanism discussed in the following is based. We want to stress that the measured force-dependencies of single pili are representative of the behaviour of pili during cell motility, as all optical tweezers experiments were done with living cells (that have the same number of pili as in the motility experiments). Tug-of-war model for twitching motility To address the question whether a tug-of-war mechanism can account for the patterns of motility observed in the experiments, we next developed an explicit stochastic tug-of-war model in two dimensions (see Fig. 3a,b and Methods). In the model, we describe the bacterium as a point particle on a planar surface, with pili emanating radially from it in random directions (the exact geometry of the cell is not modelled explicitly, because persistent motion was seen both for dumb-bell shaped diplococci and spherical monococci [15] ). The pili are described as straight rods, since the measured persistence length of 5 μm (ref. 19 ) exceeds the typical pilus length in our strain (≈1 μm, see Supplementary Table 1 ). The motion of the bacterium is determined by the (two-dimensional vectorial) balance of forces between the retracting pili (equation 3 in Methods), which accounts for the angles between the pili. In the special case where several pili extend in the same direction, the total force experienced in that direction is shared equally among these pili. The force balance equation also contains a friction term that describes the friction between the cell and the surface (see Supplementary Note 3 and Supplementary Fig. 3 ). The dynamics of the pili is described by their elongation and retraction, and their stochastic binding and unbinding from the surface. In addition, the model incorporates bundling of pili and allows pili that have fully retracted to re-elongate with a certain probability. These two aspects are discussed below. 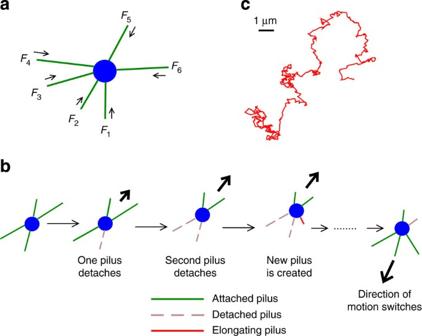Figure 3: Two-dimensional tug-of-war mechanism for twitching motility: (a) A bacterium with pili emanating in different directions. The arrows indicate the retraction of pili; the forces experienced by the pili are denoted byFiand taken as positive if they oppose the direction of retraction. (b) Basic tug-of-war mechanism: an imbalance in pulling forces in different directions is amplified by detachment of those pili that experience large force, resulting in directed motion. The direction of motion can change stochastically. (c) A typical trajectory as obtained from the simulations for the case without memory. Figure 3: Two-dimensional tug-of-war mechanism for twitching motility: ( a ) A bacterium with pili emanating in different directions. The arrows indicate the retraction of pili; the forces experienced by the pili are denoted by F i and taken as positive if they oppose the direction of retraction. ( b ) Basic tug-of-war mechanism: an imbalance in pulling forces in different directions is amplified by detachment of those pili that experience large force, resulting in directed motion. The direction of motion can change stochastically. ( c ) A typical trajectory as obtained from the simulations for the case without memory. Full size image The retraction velocity v r and the unbinding rate ε depend on the forces experienced by the pili; their force-dependence is given by the relations measured above. The force-dependent unbinding rate provides a mechanism for the stochastic selection of a direction, without the need for localization of the retraction activity: an imbalance in the number of pili pulling in opposite directions has the effect that pili on the ‘weaker side’ experience larger force and are thus more likely to unbind than the pili on the ‘strong side’. Unbinding of a pilus, however, enhances the imbalance, resulting in a cascade of unbinding and rapid motion in the direction of the pili that won the tug-of-war ( Figs 3b and 4 ). As a consequence, large forces persist only for very short times ( Fig. 4 ). The direction can be reversed stochastically, when the force balance is changed by further unbinding or rebinding of pili, by the disappearance of a pilus by full retraction or by the generation of new pili. 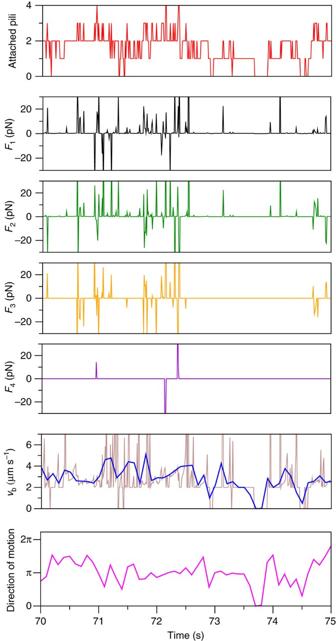Figure 4: Forces and bacterial motion in an example simulated trajectory with up to four pili. The individual panels (top to bottom) show the number of pili that are bound to the surface, the forceFiexperienced by these pili (=0 for detached pili), the velocityvbof the bacterium and the direction of bacterial motion (angle in a fixed coordinate system). Large forces are seen to be present only for short times, the same observation holds for negative forces, which arise, if two pili exert a supporting force on a third pilus in the direction of its retraction. For the bacterial velocity, we also show values averaged over a time interval of 0.1 s (blue), the time resolution of the motility experiments. Likewise, the direction data are also averaged over this time interval. Figure 4: Forces and bacterial motion in an example simulated trajectory with up to four pili. The individual panels (top to bottom) show the number of pili that are bound to the surface, the force F i experienced by these pili (=0 for detached pili), the velocity v b of the bacterium and the direction of bacterial motion (angle in a fixed coordinate system). Large forces are seen to be present only for short times, the same observation holds for negative forces, which arise, if two pili exert a supporting force on a third pilus in the direction of its retraction. For the bacterial velocity, we also show values averaged over a time interval of 0.1 s (blue), the time resolution of the motility experiments. Likewise, the direction data are also averaged over this time interval. Full size image Analysis of simulated trajectories To describe twitching motility as a tug-of-war, we generated many (~10 4 ) trajectories with model parameters estimated from experiments ( Supplementary Table 2 ), each at least 40 s long, and determined the mean square displacement δ 2 ( t ). The simulated trajectories ( Fig. 3c and Supplementary Fig. 4 ) resemble the experimental ones [15] , displaying directed motion over short time scales, but random movements over large times. This behaviour is reflected in the mean squared displacement, which exhibits a transition from a quadratic to a linear time-dependence, corresponding to directed and diffusive motion ( Fig. 5a ). The mean squared displacement was fitted with δ 2 ( t )= D eff ( t − t c [1−exp(− t / t c )]), the same function used previously to fit the experimental trajectories [15] to determine the persistence time t c and the effective diffusion coefficient, D eff = δ 2 ( t )/ t for long times t . The time-dependence of the diffusion coefficient (which approaches D eff for large times) is shown in Fig. 5b . In these plots the unknown parameters (the rebinding rate π 0 , the re-elongation probability p re and the bundling probability p bdl , see Supplementary Table 2 ) were chosen such that the persistence time and the diffusion coefficient match the observed values. With this choice of parameters, a pilus typically elongates and retracts one to two times during its lifetime, and a cell typically has one or two minibundles of two to three pili. This choice of parameters is however not unique; the conditions for agreement with the experimental trajectories are discussed below. 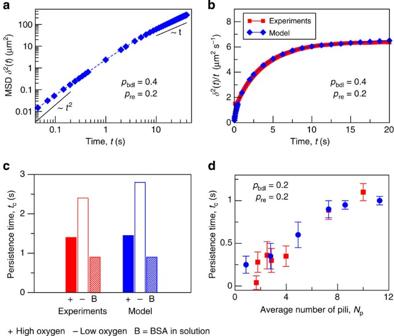Figure 5: Twitching motility in a tug-of-war model: (a) Mean squared displacementδ2(t) of simulated bacterial trajectories as a function of timet. Parameters (Supplementary Table 2) are for for wild-type bacteria with an average number ofNp≃7 pili per cell. (b) Comparison of model (blue) and experiments (red) for the time-dependent effective diffusion coefficientδ2(t)/t. (c) Persistence time for different experimental conditions: standard aerobic, anaerobic (reduced velocity) and aerobic in the presence of excess BSA (reducing bundling). The latter two conditions are described in the model by the standard parameters with a reduced retraction velocity (vr=1 μm s−1) or a reduced bundling probability (pbdl=0.2, respectively). (d) Dependence of the persistence timetcon the number of pili per cell (blue: model, red: experimental data for the strain with induciblepilE15, error bars: s.e. values from correlated random walk fit). The bundling probability ispbdl=0.2 in this plot to mimic the effect of excess BSA present in these experiments (seeSupplementary Note 4). Figure 5: Twitching motility in a tug-of-war model: ( a ) Mean squared displacement δ 2 ( t ) of simulated bacterial trajectories as a function of time t . Parameters ( Supplementary Table 2 ) are for for wild-type bacteria with an average number of N p ≃ 7 pili per cell. ( b ) Comparison of model (blue) and experiments (red) for the time-dependent effective diffusion coefficient δ 2 ( t )/ t . ( c ) Persistence time for different experimental conditions: standard aerobic, anaerobic (reduced velocity) and aerobic in the presence of excess BSA (reducing bundling). The latter two conditions are described in the model by the standard parameters with a reduced retraction velocity ( v r =1 μm s −1 ) or a reduced bundling probability ( p bdl =0.2, respectively). ( d ) Dependence of the persistence time t c on the number of pili per cell (blue: model, red: experimental data for the strain with inducible pilE [15] , error bars: s.e. values from correlated random walk fit). The bundling probability is p bdl =0.2 in this plot to mimic the effect of excess BSA present in these experiments (see Supplementary Note 4 ). Full size image We next compared the persistence times for different experimental conditions. Experimentally, we reduced the speed of pilus retraction by a factor of 2 by introducing anaerobic conditions ( Fig. 2f and ref. 36 ). In these experiments, the speed switches very abruptly upon rapid oxygen depletion, so that the surface properties of the cell are likely to remain unchanged over the course of these experiments. Here, we found that the persistence time of the trajectories is increased 1.6-fold ( Supplementary Table 3 and Fig. 5c ). When we used the force–velocity relation measured for low oxygen conditions ( Fig. 2f ) in our simulations, we indeed obtained increased persistence times in good agreement with the experimental ones (open bars in Fig. 5c ). Furthermore, we added excess BSA to the solution, since this has been shown to suppress bundling of pili [26] . Under these conditions the persistence time of the experimental trajectories was reduced to 0.9 s ( Supplementary Table 3 and Supplementary Note 4 ). This reduction can be reproduced in our simulations by a smaller bundling probability ( p bdl =0.2 instead of 0.4, Fig. 5c ). Finally, we simulated bacteria with different numbers of pili by varying the pilus creation rate (see Methods for a detailed description) and determined the persistence time as a function of the average number of pili ( Fig. 5d ). Experimentally, the variation of the pilus number (achieved by controlling the pilE gene with an inducible promoter) was found to result in a strong increase of the persistence time with increasing pilus number (an approximately fourfold increase from 2 pili to 10 pili) [15] . In our simulations, we also find a pronounced increase of the persistence time with increasing pilus number, in quantitative agreement with the experimental results. A memory requirement for two-dimensional persistent motion Next, we systematically varied those parameters that have not been determined experimentally to study the requirements for persistent motion in our model. The rebinding rate π 0 of a detached pilus had a weak effect on the persistence time (except for very small π 0 , where the persistence time was strongly reduced, see Supplementary Fig. 5a ) and was thus set to a sufficiently large constant value ( Supplementary Table 2 ). Varying the bundling probability and the re-elongation probability, we found a range of parameters for which the persistence time for wild-type bacteria with N p ≃ 7 pili was consistent with the experimental value of ≃ 1.4 s. This range is shown as the green area in Fig. 6a and contains the parameters used above (indicated by the star) as well as cases without bundling ( p bdl =0) or without re-elongation ( p re =0), see also Supplementary Fig. 5b–e . Re-elongation alone can however not fully explain the experimental data, as the effective diffusion coefficient is underestimated and the effect of excess BSA is unclear ( Supplementary Fig. 5c,e ). By contrast, in the absence of both bundling and re-elongation, the persistence time is smaller (0.6 s) than the experimental value. Likewise, a strong increase of the persistence time with the pilus number N p , in agreement with the experimental result, was found for both bundling and re-elongation ( Fig. 5d ) as well as only bundling or re-elongation, but not in the absence of both (black circles in Fig. 6b and Supplementary Fig. 5d ). 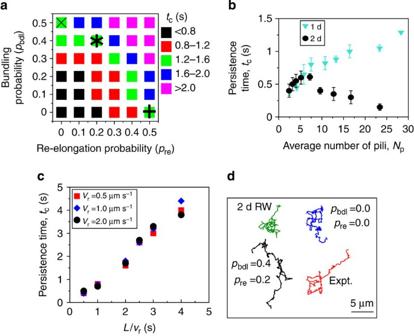Figure 6: Requirement for memory: (a) Dependence of the persistence timetcon the bundling probabilitypbdland on the re-elongation probabilitypre(for WT). In the green region,tcis consistent with the experiments. The star indicates our preferred parameter combination (which provides good agreement with the experimental data also for the effective diffusion coefficient, seeFig. 5b). The cross and the plus indicate the two parameter combinations used to study bundling and re-elongation separately (Supplementary Fig. 5). (b) Tug-of-war in one and two dimensions: Persistence time (fitted parameter value±s.e.) as a function of the number of pili in the case without memory (pbdl=pre=0, black circles) and a one-dimensional version of the model, where pili are only generated at angles 0° and 180° (cyan triangles). The persistence time is found to increase with increasing pilus number in one-dimension, while in the two-dimensional model it decreases for large pilus numbers (black circles). (c) In the absence of a mechanism for memory (pbdl=pre=0), the persistence time is strongly correlated to and limited byL/vr, the ratio of average pilus length and retraction velocity, which represents the typical time required for a full retraction of a pilus. (d) Typical trajectories with and without memory (additional trajectories are shown inSupplementary Fig. 4). Forpbdl=pre=0 (blue), the trajectories resemble those of a simple two-dimensional random walk with step size equal to the average pilus length (2d RW, green). In the model with bundling and re-elongation (black) as well as in the experimental trajectories (red), the cells move in the same direction over longer distances. Figure 6: Requirement for memory: ( a ) Dependence of the persistence time t c on the bundling probability p bdl and on the re-elongation probability p re (for WT). In the green region, t c is consistent with the experiments. The star indicates our preferred parameter combination (which provides good agreement with the experimental data also for the effective diffusion coefficient, see Fig. 5b ). The cross and the plus indicate the two parameter combinations used to study bundling and re-elongation separately ( Supplementary Fig. 5 ). ( b ) Tug-of-war in one and two dimensions: Persistence time (fitted parameter value±s.e.) as a function of the number of pili in the case without memory ( p bdl = p re =0, black circles) and a one-dimensional version of the model, where pili are only generated at angles 0° and 180° (cyan triangles). The persistence time is found to increase with increasing pilus number in one-dimension, while in the two-dimensional model it decreases for large pilus numbers (black circles). ( c ) In the absence of a mechanism for memory ( p bdl = p re =0), the persistence time is strongly correlated to and limited by L / v r , the ratio of average pilus length and retraction velocity, which represents the typical time required for a full retraction of a pilus. ( d ) Typical trajectories with and without memory (additional trajectories are shown in Supplementary Fig. 4 ). For p bdl = p re =0 (blue), the trajectories resemble those of a simple two-dimensional random walk with step size equal to the average pilus length (2d RW, green). In the model with bundling and re-elongation (black) as well as in the experimental trajectories (red), the cells move in the same direction over longer distances. Full size image This result was surprising, because work on one-dimensional tug-of-war models in the context of cytoskeletal transport [8] had suggested that a strong dependence on the number of motors was a generic feature of tug-of-war model. We thus tested a one-dimensional version of our present model, where pili are only generated at the poles of the bacterium. This model also exhibited a pronounced increase of the persistence time with increasing number of pili, in contrast to the two-dimensional model ( Fig. 6b ). Moreover, simulations of the two-dimensional model with different pilus lengths L and different retraction velocities v r show that in the absence of bundling and re-elongation, the persistence time t c is strongly correlated with L / v r . This quantity provides an estimate of the typical time it takes for a pilus to retract completely ( Fig. 6c ). The latter observation suggests that the full retraction of a pilus results in the loss (or randomization) of the direction of motion, such that the time L / v r limits the persistence time. This effect is only seen in the two-dimensional case, where the direction of motion can be changed incrementally, but not in one dimension, where a sharp reversal is required. Both bundling and re-elongation provide mechanisms for a memory of the direction of motion beyond the retraction of a single pilus, by making it likely that another retraction (of either the same or another pilus) will occur in the same direction (in the case of bundling, this effect requires that pili in a bundle elongate and retract independently, see Methods). Such memory is required to reproduce two key experimental observations, persistent motion over longer distances exceeding the pilus length and the pronounced increase of the persistence time with increasing pilus number. The qualitative effect of such memory is illustrated by typical trajectories in Fig. 6d (additional trajectories are shown in Supplementary Fig. 4 ), where for comparison we also show a simple 2d-random walk with step size given by the average pilus length and an experimental trajectory. Experimental test of memory in type IV pilus retraction As the tug-of-war without memory cannot quantitatively explain the experimental data, we searched for experimental evidence of memory. Transmission electron microscopy (TEM) images of the bacteria often showed minibundles consisting of two to three pili ( Fig. 7a,b and Supplementary Fig. 6 ). Typical numbers of such bundles per cell were one or two. These numbers are consistent with the numbers obtained by matching our model to the motility data. Furthermore, we assessed whether pilus retractions were correlated in time. To that end, we measured the distribution of time intervals τ between two subsequent retraction events as obtained from laser tweezers experiments ( Fig. 7c ). We found that the distribution was inconsistent with a single-exponential distribution ( Fig. 7d ), suggesting that retractions may occur in ‘bursts’. To further analyse these bursts, we considered temporal correlations between retraction events. If there was an enhanced probability for pilus retraction at a certain location for a certain time (due to the presence of either a bundle of pili or a single pilus that is regrown several times), the time intervals τ between several consecutive retractions should be significantly shorter than the average time interval between retractions. Therefore the deviation from the average should show temporal correlations. This would correspond to the assumption that the probability for a retraction is increased after another retraction has occurred. We therefore numbered the retraction events in an experimental trajectory consecutively with respect to a reference retraction. We denote by τ ( R ) the time interval between retraction events with numbers R and R +1. We then analysed the temporal correlation coefficient . We found that there was a significant correlation between several (~10) subsequent retractions ( Fig. 7e ), indicating temporal correlation of type IV pilus retraction. These experiments confirm that pilus dynamics has memory. 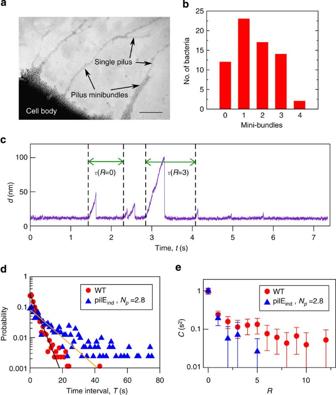Figure 7: Experimental evidence for memory effects. (a) Typical TEM image ofN. gonorrhoeaeshowing individual pili and pilus minibundles (scale bar, 200 nm). (b) Histogram of the number of bundles per cell as seen from images like in (a) (n=68 bacteria). (c) Typical time course of pilus retractions in laser tweezers experiments: Binding of a pilus to a bead and subsequent retraction of the pilus lead to a deflectiondof the bead from the centre of the laser trap until the pilus detaches again. The interval between retraction events are denoted byτand numbered consecutively (with indexR) relative to a reference retraction event. The deflection data have been smoothed over 20 data points. (d) Distribution of time intervals between pilus retractions for wild-type cells (red) and thepilE-inducible strain with 0.25 mM IPTG, corresponding toNp=2.8 pili per cell (blue);n>500 retractions for each condition. An exponential fit is inconsistent with the tail of long time interval. (e) Correlation coefficientof the time intervals τ between retraction events as a function of the numberRof separating retraction events for the same data as (d). The error bars show s.e. values of the correlation function. Figure 7: Experimental evidence for memory effects. ( a ) Typical TEM image of N. gonorrhoeae showing individual pili and pilus minibundles (scale bar, 200 nm). ( b ) Histogram of the number of bundles per cell as seen from images like in ( a ) ( n =68 bacteria). ( c ) Typical time course of pilus retractions in laser tweezers experiments: Binding of a pilus to a bead and subsequent retraction of the pilus lead to a deflection d of the bead from the centre of the laser trap until the pilus detaches again. The interval between retraction events are denoted by τ and numbered consecutively (with index R ) relative to a reference retraction event. The deflection data have been smoothed over 20 data points. ( d ) Distribution of time intervals between pilus retractions for wild-type cells (red) and the pilE -inducible strain with 0.25 mM IPTG, corresponding to N p =2.8 pili per cell (blue); n >500 retractions for each condition. An exponential fit is inconsistent with the tail of long time interval. ( e ) Correlation coefficient of the time intervals τ between retraction events as a function of the number R of separating retraction events for the same data as ( d ). The error bars show s.e. values of the correlation function. Full size image Next, we addressed the question whether the reduction of the average number of pili per cell affected bursting of pilus retractions, using the pilE -inducible strain with an average number of N p =2.8 pili per bacterium. As for wild type, the distribution of time intervals τ between two subsequent retraction events deviated strongly from an exponential distribution ( Fig. 7d ). Furthermore, we found that time intervals were correlated for three consecutive retractions ( Fig. 7e ). Taking into account the average time intervals (1.3 s for wild type and 10 s for the pilE ind mutant), significant correlation was observed for times on the order of 13 and 30 s, respectively. For the pilE ind strain, we observed a single bundle only in 7% of all cells imaged by TEM, in agreement with earlier reports showing that gonococcal strains with a reduced number of pili revealed significantly less bundles [34] . We therefore conclude that the characteristic time scale at which bursts of pilus retractions occur exceeds 10 s independent of pilus bundling. Instead we propose that re-elongation of pili is important for temporal persistence. The fact that we do not see highly persistent movement of gonococci at reduced pilus number is due to the fact that with an average of 2.8 pili per cell, the simultaneous attachment of more than one pilus, and thus cooperation of pili, is unlikely. In this study we have addressed the mechanism by which the retraction of pili is coordinated during twitching motility of peritrichously piliated bacteria using N. gonorrhoeae as a model system. Specifically, we addressed the question whether the pili could be coordinated through the mechanical forces that pili exert on each other. We have developed a two-dimensional tug-of-war model based on the experimental characterization of the dynamics of individual pili. Unexpectedly, we found that the two-dimensional tug-of-war is less efficient in generating persistent motion than the one-dimensional tug-of-war studied previously in the context of cytoskeletal transport [8] . The systematic comparison of the patterns of motility obtained for different variants of the model with the corresponding experimental data showed that a form of directional memory is required to explain key experimental observations, in particular (i) persistent motion over lengths exceeding the length of a single pilus and (ii) the pronounced increase in persistence time with increasing number of pili per cell as observed in mutants with inducible pilE . Our model contains two mechanisms for such memory, that are not mutually exclusive, the alignment of pili in the same direction in minibundles and re-elongation of a pilus after complete retraction. Experiments gave evidence for formation of minibundles under our experimental conditions and our experiments with excess BSA indicate that these bundles enhance persistence. However, memory was observed even under conditions where bundling was unlikely, strongly suggesting a key role for pilus re-elongation. We interpret re-elongation to reflect the presence of a core complex at the base of the pilus that is stable and immobile in the membrane for a time scale longer than the retraction of a single pilus. This complex most likely consists of the inner membrane protein PilG, the outer membrane channel PilQ and periplasmic elements. Binding of the elongation ATPase PilF and of the retraction ATPase PilT is likely to be dynamic, so that re-elongation may be induced by the rebinding of PilF to the core complex. This interpretation is consistent with observations in M. xanthus showing the presence of a stable complex spanning the inner and outer membranes in the absence of the pilus filament [29] , [37] and stable localization at the cell poles of the PilQ and the PilG homologues, while PilT localization is dynamic [28] . All things considered, our theoretical and experimental results suggest that re-elongation from membrane-standing complexes that are stable for several seconds is sufficient for generating persistent motion and that persistence is enhanced by small pilus bundles. Importantly, our minimal model does not require biochemical regulation of the localization of the ATPases PilT and PilF for describing the experimental data, in contrast to M. xanthus [38] . In summary, we have shown by a combination of experimental and theoretical methods that twitching motility in N. gonorrhoeae is coordinated by a tug-of-war with directional memory. The increased persistence of the movements arising from such a directional memory increases the effective diffusion coefficient with which the bacteria explore a surface, and thus the surface range that they explore, likely facilitating surface colonization. In contrast to, for example M. xanthus , where type IV pili power directed chemotactic motion [39] , the genome of N. gonorrhoeae does not reveal chemotactic systems [40] , but twitching motility could be guided along certain directions by clues on the surface that modulate adhesion strength. For example, it has been shown that the fluidity of a surface affects the persistence of the motion [41] and fluidity is likely to vary on the surface of host cells. On the part of the bacterium, motility can be regulated by mechanisms that modulate either the pilus number, for example, through transcriptional regulation of the pilin promoter [42] , or the strength of adhesion, for example, via post-translational modifications of the pilus surface [43] , [44] . These control mechanism may play a role during infection or during biofilm formation. For example, it was recently shown for N. gonorrhoeae that both pilus bundling and the persistence time of motility are strongly reduced by seminal plasma, demonstrating indeed that the transmission conditions affect motility at the level of directional persistence [45] . Overall, type IV pili are essential for two opposing phenotypes in N. gonorrhoeae , namely for motility and for clustering. Directional persistence is likely to bias the behaviour towards motility. Finally, from a more general point of view, our results also point towards the importance of mechanical coordination for biological regulation. Bacterial culture and strains We used the N. gonorrhoeae strains N 400, an opa− selected recA -inducible strain [46] , and an isogenic strain, pilE ind , which carried the pilE gene under the control of an IPTG-inducible promoter [47] . Bacteria were maintained on agar containing 5 g l −1 NaCl (Roth), 4 g l −1 K 2 HPO 4 (Roth), 1 g l −1 KH 2 PO 4 (Roth), 15 g l −1 protease peptone No. 3 (BD), 0.5 g l −1 starch (Sigma Aldrich) and 10 ml l −1 IsoVitaleX enrichment (BD) and were grown overnight at 37 °C and 5% CO 2 . IPTG was added to the plates and to the cell culture medium for microscopy as required. Experimental characterization of twitching motility N. gonorrhoeae were suspended in cell culture medium containing phenol-red free DMEM (Gibco) with 2 mM L -glutamine (Gibco), 8 mM sodium pyruvate (Gibco), 5 mM ascorbic acid (Roth) and 30 mM HEPES (Roth), and applied to treated glass coverslides. Glass coverslides were washed in 1 M KOH for 10 min, rinsed with Milli-Q and dried under a nitrogen stream. For BSA coating the coverslides were subsequently incubated with a BSA solution (10 mg ml −1 in Milli-Q) for 30 min, washed again with Milli-Q and dried with nitrogen. For microscopy, bacteria were suspended in cell culture medium containing phenol-red free DMEM (Gibco) with 2 mM L -glutamine (Gibco), 8 mM sodium pyruvate (Gibco), 5 mM ascorbic acid (Roth) and 30 mM HEPES (Roth), applied to the coverslide and sealed. Movies were recorded at a rate of 10 frames per second for 2 min. Individual motile bacteria were tracked with pattern matching capabilities built into National Instruments Labview 7:1, St Andrews Tracker 1:0:2 provided by Graham Milne (see also refs 15 , 36 ). For the experiments under anaerobic conditions, an oxygen scavenger consisting of the enzyme protocatechuate-3,4-dioxygenase and the substrate protocatechuic acid was added that depleted oxygen within 2 min (ref. 36 ). Speed switching occurred within seconds in response to oxygen depletion. Thus, we consider it as highly unlikely that the surface structures (or any cell properties that require protein synthesis and might be induced by the anaerobic conditions) change within this short period of time. Characterization of single pilus retraction speed and unbinding times For measuring the speed generated by a single retracting pilus at a well-defined force, we used a previously described laser tweezers setup ( Fig. 2a,b ) [48] . Pilus retraction was analysed in the same media as twitching motility. In short, a bead was trapped and approached to the bacterium that was fixed to a polystyrene coated glass slide while the entire sample was mounted on a piezo stage (see Fig. 2a ) [48] . The trapped bead was imaged directly onto a four-quadrant photo diode, allowing to monitor the displacements with high spatial and temporal resolution. The piezo stage was actuated by a computer-controlled force feedback loop to record single pilus dynamics at constant force. When a single pilus bound and retracted, it deflected the bead from the centre of the laser trap. For constant force, the displacement of the bead due to a pilus retraction was allowed to reach a certain threshold, at which the force clamp was triggered. Hereafter, the displacement and hence the force was kept constant by moving the piezo stage with the bacterium relative to centre of the optical tweezers. The movement of the bacterium is a direct measure of the pilus length change. To determine stalling forces, this setup was used without force feedback. The force–velocity relation was measured with carboxylated polystyrene beads with 2 μm in diameter (Kisker Biotech, Steinfurt, Germany). The corresponding data in Fig. 2f are a combination of previously published data [36] and newly acquired data ( Supplementary Fig. 2 ). For measuring the unbinding times of single pili from a BSA-treated glass surface, we used BSA-treated silica beads for the laser tweezers assay. The unbinding time was defined as the time period between reaching the clamp force and the breaking of the pilus from the bead ( Fig. 2c ). Construction of the model Our tug-of-war model describes the bacterium as a point object on a planar surface, characterized by a position (the shape of the bacterium is not described explicitly, because persistent motion with similar persistence time has been observed for different shapes, specifically diplococci and gonococci [15] ). Pili are described by their length L i and direction (two-dimensional unit vector ) and their internal state (bound to the surface, unbound or elongating). Switching between these states is described stochastically with the rates given in the main text. The rate for unbinding of a pilus, ε ( F i ), depends on the force F i experienced by the pilus. By F i we denote the force along the direction of the pilus, which we take as positive if it opposes the pilus’ retraction, that is, if . Pilus retraction and movements of the bacterium are described by deterministic dynamics. The retraction of bound and unbound pili is described by Newly created pili grow with d L i /d t = v e and the movement of the bacterium is given by d x b /d t = v b . For unbound pili, the forces F i are 0. The forces F i for bound pili as well as the velocity of the bacterium are determined from two conditions: (i) the force balance which includes sharing of forces by pili extending in the same direction and where γ is the friction coefficient of the bacterium; and (ii) and the requirement that all length changes of bound pili are consistent with the movement of the bacterium, The latter equation is derived in the following way: during a time interval Δ t , the length of a pilus changes due to retraction from L i to L i − v ( F i )Δ t . The new length of the pilus can also be expressed by the distance between the attachment point of the pilus on the surface (which has not changed), x b + L i e i , and the position of the bacterium which has changed from x b to x b + v b Δ t . Equating the two expressions leads to Equation 4. Simulations Simulations were performed with a discrete-time Monte-Carlo-type algorithm. At every time step (chosen to be Δ t =10 −4 s, which is much smaller than the experimental resolution of ~10 −1 s), all the pili are updated with probabilities corresponding to the rates of first attachment, unbinding and rebinding attempt. In addition, a new pilus is created with probability c Δ t . A newly created pilus has length 1 nm corresponding to the length of a single monomer. Its direction is chosen randomly with a uniform distribution between 0 and 2π; this distribution is modified in the presence of bundles ( p pdl >0), as explained below. The angle of the pilus can change during integration of the spatial dynamics. To mimic a fixed position of a pilus on the surface of a bacterium, for which changes of the angle correspond to bending of the pilus with a certain rigidity rather than floating on that surface, we restore the angle to its initial value when a pilus detaches. After these stochastic events, the forces on the bound pili are calculated using the force balance equation, Equation 3. Then the position of the bacterium and the lengths are updated according to Equation 3 and Equation 2 respectively. Pili retracting to a length L i ≤0, that is, being fully retracted into the cell body, are assumed to release from the surface (in principle they could remain attached with a tip still present on the cell surface, but would detach spontaneously within ~1 s). A fully retracted pilus may re-elongate with probability p re , otherwise it is removed from the description. Pili are described as straight rods in model, since the measured persistence length of a pilus (5 μm (ref. 19 )) is longer than the average pilus length in our strains (≈1 μm, see Supplementary Table 1 ). Thus, upon re-elongation a pilus points in exactly the same direction as before full retraction (it may however attach and start retracting at a different length). This idealization should be taken as representing a pilus that attaches at a location nearby that straight line. The re-elongation probability p re is expected to depend on the concentration of the pilus subunits, which is varied in the experiments with inducible pilE . We therefore coupled it to the creation rate c of new pili through p re =1/(1+ ηc WT / c ), where c WT is the creation rate for wild-type cells and . Re-elongation of a pilus can be expected to occur if proteins at the base of a pilus remain assembled and localized at the same position on the cell surface for a time longer than a single retraction. Bundling is mimicked by a bundling probability p bdl . When a new pilus is generated, its direction is aligned with the direction of a pilus that is already present with probability p bdl n p / n WT , where n p is the number of pili present at that moment (normalized to the average number in wild-type cells), with probability (1− p bdl n p / n WT ), the direction is chosen randomly (this probability was not reduced below 0.1 to ensure some pili are always directed randomly). In our model, bundles are idealized in the sense that retraction and elongation of pili in a bundle are independent of each other, that is, the retraction of one pilus is not slowed down or blocked by the other pili in the bundle. Thus, we assume that the interactions between the pili are weak. With stronger interactions, retractions of different pili in a bundle may interfere with each other and the positive effect of bundles of the persistence time of the trajectories would be reduced. Our implementation of pilus bundles can also be used for pili that are not bound to each other (no actual interactions between the appendages), but that emerge from a cluster of pilus assembly proteins in the membrane, so that they emanate in the same direction. This situation is however not suggested by the TEM images. The forces experienced by the bound pili are re-calculated twice per time step, before carrying out the stochastic events and before integrating the spatial dynamics. In contrast to the one-dimensional tug-of-war model for cytoskeletal motors studied earlier [8] , [35] , the forces (and thus the force-dependent rates) vary over time in a continuous fashion, as the angles of the pili change during the motion. This is the main reason why a discretized time is used in the simulations. In the experiments, bacteria start twitching immediately after coming in contact with the surface. In simulations we use similar initial conditions. Every trajectory starts with a random number of initial pili (≤7). We let the bacterium move for an initial period of ≈5 s, after which data are collected for at least 40 s. How to cite this article: Marathe, R. et al. Bacterial twitching motility is coordinated by a two-dimensional tug-of-war with directional memory. Nat. Commun. 5:3759 doi: 10.1038/ncomms4759 (2014).